Family-wide analysis of poly(ADP-ribose) polymerase activity The poly(adenosine diphosphate (ADP)-ribose) polymerase (PARP) protein family generates ADP-ribose (ADPr) modifications onto target proteins using NAD + as substrate. Based on the composition of three NAD + coordinating amino acids, the H-Y-E motif, each PARP is predicted to generate either poly(ADPr) (PAR) or mono(ADPr) (MAR). However, the reaction product of each PARP has not been clearly defined, and is an important priority since PAR and MAR function via distinct mechanisms. Here we show that the majority of PARPs generate MAR, not PAR, and demonstrate that the H-Y-E motif is not the sole indicator of PARP activity. We identify automodification sites on seven PARPs, and demonstrate that MAR and PAR generating PARPs modify similar amino acids, suggesting that the sequence and structural constraints limiting PARPs to MAR synthesis do not limit their ability to modify canonical amino-acid targets. In addition, we identify cysteine as a novel amino-acid target for ADP-ribosylation on PARPs. The primary function of the 17-member poly(adenosine diphosphate (ADP)-ribose) polymerase (PARP) protein family is to generate ADP-ribose (ADPr) modifications onto target proteins using NAD + as substrate [1] . The best understood PARP functions involve poly(ADPr) (PAR) synthesis and include physiological functions in cell division [2] , [3] , [4] , [5] , [6] , transcriptional regulation (reviewed in ref. 7 ) and regulation of protein degradation [8] , [9] . PAR also functions during cell stress responses such as DNA damage [10] , heat shock [11] , [12] and the cytoplasmic stress response [13] . Recently, it was shown that certain PARPs, such as PARP10 and PARP14, only generate mono(ADPr) (MAR) [14] . However, it is not clear if other PARP family members are also limited to MAR synthesis. Computational analysis of amino-acid sequence in combination with this data led to the prediction that each PARP can generate either PAR or MAR, but not both [14] . The functional distinction between PAR and MAR synthesis is important since the type of ADPr modification generated has critical impacts on the potential mechanisms of function. MAR modifications add single ADPr units onto proteins whereas PAR polymers can be up to 200 units in length when generated in vitro , and can contain both linear and branched glycosidic linkages [15] . Although both can regulate the function of target proteins via direct covalent modification, PAR can also recruit binding proteins that contain a 20-amino acid PAR binding motif [16] as well as characterized PAR binding domains including Macro [17] , PBZ [18] and WWE [19] domains. This allows PAR to function as a reversible high-density protein binding scaffold for the nucleation of multiprotein complexes of great complexity. Therefore, identifying the type of ADPr modifications generated by each PARP is critical to understanding specific mechanisms of PARP function. Although less is known about MAR, our recent family-wide analysis of PARP function and previous work by other labs has identified important functions for PARPs predicted to generate MAR. These include regulation of transcription (PARP3, 7 and 14) [20] , [21] , [22] , signal transduction pathways (PARP10 and 14) [23] , [24] , [25] , the unfolded protein response (PARP16) [26] , the actin cytoskeleton (PARP14) [27] , and membrane organelles (PARP8 and 16) [27] . The diversity of pathways that appear to be regulated by MAR demonstrates the general importance of MAR in cell function and suggests that a deeper understanding of the molecule is in order. The primary predictors of PARP enzymatic activity are thought to be the amino acids that catalyse the ADPr transfer reaction. The PARP catalytic domain contains a signature H-Y-E motif originally identified in various bacterial mono-ADP-ribosyltransferase toxins that also mediate ADPr transfer. Histidine and tyrosine residues are required for binding of the substrate NAD + and the glutamate for catalysis [28] , [29] . 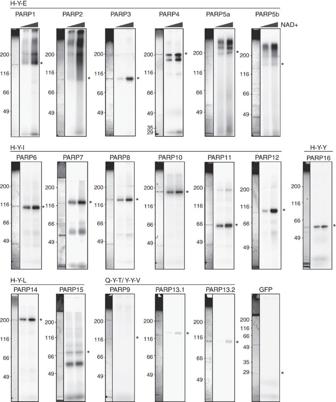Figure 1: H-Y-E motif is not the sole indicator for PAR synthesis activity. GFP–PARPs were immunoprecipitated from 293F cells and subjected to NAD+incorporation reactionsin vitrowith 5 or 10 μM cold NAD+supplemented with a constant ratio of32P-NAD+. Automodifed PARPs were resolved on SDS–PAGE gels and subjected to autoradiography. Representative Coomassie stained gels for each PARP purification are shown to the left of the autoradiogram and the expected molecular weight of the PARP indicated by an asterisk. Assays were repeated at least twice. Of the H-Y-E motif containing PARPs, PARP1, 2, 5a and 5b generated polymer, as evidenced by the smear of signal starting from the molecular weight of the PARP. The remaining PARPs resolve as a discreet band, indicating that they do not generate poly(ADPr). See alsoSupplementary Figs 1–3. Since most PARPs contain an isoleucine, leucine or tyrosine in place of the catalytic glutamate they are predicted to generate MAR [14] ( Supplementary Table 1 ). In addition, PARP9 and 13 also contain amino-acid substitutions for the NAD + binding histidine and are predicted to be inactive [14] . Secondary structural features of the PARP catalytic domain are also predicted to influence catalytic activity. In addition to the NAD + binding residues of the H-Y-E motif, the Donor loop (D-loop) shapes the substrate binding pocket and interacts with NAD + (ref. 30 ). This loop varies in size and rigidity within the PARP family and analysis of the binding of small molecule PARP inhibitors to PARP catalytic domains identified the D-loop as a structural element that contributes to differential inhibitor binding [30] . Therefore, the shape of the substrate binding pocket, partly lined by the D-loop, could contribute to differences in NAD + binding among the PARPs and impact catalytic activity or enzyme kinetics. Another structural component of the PARP catalytic domain is the acceptor pocket, partly lined by the loop between β sheets 4 and 5 and referred to as the acceptor loop. This loop is implicated in the binding of either protein substrate or ADPr acceptor for bacterial mono-ADP-ribosyltransferases or eukaryotic PARPs, respectively and varies in length among PARP proteins [14] , [31] , [32] , [33] . Therefore, the ability to bind to an incoming ADPr unit on a PAR polymer could vary based on the structure of the acceptor loop, impacting the ability to elongate a PAR chain or create a branched modification. Whether or not these amino acid or structural constraints thought to limit PARP activity to MAR synthesis affect selectivity of amino-acid targets is unknown. Most current data pertaining to amino-acid selectivity is based on the PAR generating PARP1; however, even here, amino-acid selectivity is unclear. Although most studies identify glutamate and aspartate residues as the primary targets of modification [34] , [35] , [36] , [37] , lysines have also been identified [38] , [39] . Here we take a systematic approach to examine PARP enzymatic activity, assaying automodification of each member of the PARP family of proteins with high resolution. Our results suggest that the primary enzymatic activity for the PARPs is MAR synthesis and that the amino-acid identity of the H-Y-E motif is not the sole indicator of PAR or MAR synthesis. They further demonstrate that MAR and PAR generating PARPs modify both acidic amino acids and lysines and identify ADPr modifications on cysteine residues of PARPs. In conjunction with our recent work identifying new PARP functions from a PARP family-wide analysis, these results demonstrate the importance of MAR as a product of PARP activity as the majority of PARP phenotypes result from knockdown of MAR-generating PARPs [27] . PARP enzymatic activity assays Recent work has provided experimental evidence demonstrating PAR or MAR activity for several of the PARPs ( Supplementary Table 1 ). The most commonly used approach has been resolution of automodified PARPs on SDS–PAGE gels [13] , [14] , [22] , [26] , [40] , [41] , [42] , [43] , [44] , [45] , [46] , [47] . PARPs that appear as distinct bands are identified as MARylating, and those that resolve as smears due to heterogeneity of attached polymers are identified as PARylating ( Supplementary Table 1 ). One problem with this approach is that it cannot distinguish between the addition of single ADPr units or addition of short oligomers of ADPr since each ADPr unit adds only 0.6 kDa to a protein and protein resolution on SDS–PAGE is both mass and charge dependent making resolution of small modifications unpredictable. To provide a more accurate analysis of PARP reaction products, we expressed and purified each full-length PARP as amino-terminal GFP fusions in human 293F cells, then performed standard automodification assays [48] previously shown to effectively measure enzymatic activity since the majority of PARP activity is self-directed [49] . Three approaches were used to analyse the reaction products: standard PAGE based automodification assays ( Fig. 1 ), hydrolysis with enzymes specific for PAR or MAR and chemical treatments to release ADPr modifications at the site of protein linkage ( Figs 2 , 3 ). The released products generated by approach 2 and 3 were then analysed using high-resolution TBE–acrylamide sequencing gels or thin layer chromatography (TLC) ( Figs 2 , 3 ). Figure 1: H-Y-E motif is not the sole indicator for PAR synthesis activity. GFP–PARPs were immunoprecipitated from 293F cells and subjected to NAD + incorporation reactions in vitro with 5 or 10 μM cold NAD + supplemented with a constant ratio of 32 P-NAD + . Automodifed PARPs were resolved on SDS–PAGE gels and subjected to autoradiography. Representative Coomassie stained gels for each PARP purification are shown to the left of the autoradiogram and the expected molecular weight of the PARP indicated by an asterisk. Assays were repeated at least twice. Of the H-Y-E motif containing PARPs, PARP1, 2, 5a and 5b generated polymer, as evidenced by the smear of signal starting from the molecular weight of the PARP. The remaining PARPs resolve as a discreet band, indicating that they do not generate poly(ADPr). See also Supplementary Figs 1–3 . 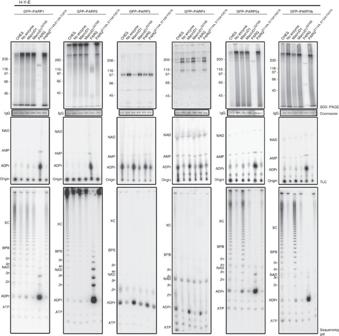Figure 2: Enzymatic and chemical release of H-Y-E PARPs indicates that additional features of PARP catalytic domain impact to enzymatic activity. Automodified PARPs were treated with CHES or the indicated wild type and catalytically inactive ADPr hydrolytic enzyme. Signal remaining attached to protein was analysed by SDS–PAGE (top row), Coomassies of either IgG (PARPs 1, 2, 5a and 5b) or PARP (PARP3 and 4) are shown below. Released product was analysed by TLC (middle row) and sequencing gel (bottom row). Assays were repeated at least twice. PARPs 1, 2, 5a and 5b release PAR ladders upon CHES treatment and are sensitive toT. curvataPARG hydrolysis. In contrast, PARP3 and 4 release ADPr upon CHES, MacroD1 andT. curvataPARG treatment, indicative of MAR synthesis activity. See alsoSupplementary Fig. 4. Full size image Figure 2: Enzymatic and chemical release of H-Y-E PARPs indicates that additional features of PARP catalytic domain impact to enzymatic activity. Automodified PARPs were treated with CHES or the indicated wild type and catalytically inactive ADPr hydrolytic enzyme. Signal remaining attached to protein was analysed by SDS–PAGE (top row), Coomassies of either IgG (PARPs 1, 2, 5a and 5b) or PARP (PARP3 and 4) are shown below. Released product was analysed by TLC (middle row) and sequencing gel (bottom row). Assays were repeated at least twice. PARPs 1, 2, 5a and 5b release PAR ladders upon CHES treatment and are sensitive to T. curvata PARG hydrolysis. In contrast, PARP3 and 4 release ADPr upon CHES, MacroD1 and T. curvata PARG treatment, indicative of MAR synthesis activity. See also Supplementary Fig. 4 . 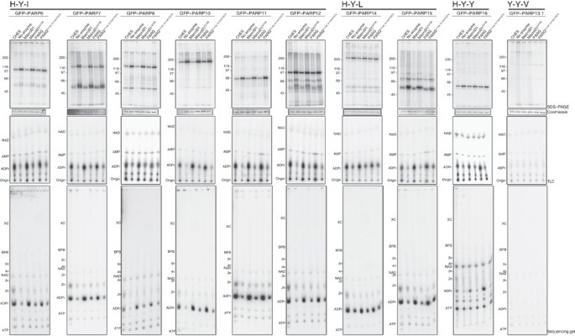Figure 3: Enzymatic and chemical release shows that MAR synthesis is the primary activity of non-H-Y-E PARPs. Automodified PARPs were treated with CHES or the indicated wild type and catalytically inactive ADPr hydrolytic enzyme. Signal remaining attached to protein was analysed by SDS–PAGE (top row), Coomassies for each PARP are shown below. Released product was analysed by TLC (middle row) and sequencing gel (bottom row). Assays were repeated at least twice. CHES, MacroD1 andT. curvataPARG treatment of non-H-Y-E PARPS results in ADPr release, indicative of MAR synthesis activity. See alsoSupplementary Figs 4,5. Full size image Figure 3: Enzymatic and chemical release shows that MAR synthesis is the primary activity of non-H-Y-E PARPs. Automodified PARPs were treated with CHES or the indicated wild type and catalytically inactive ADPr hydrolytic enzyme. Signal remaining attached to protein was analysed by SDS–PAGE (top row), Coomassies for each PARP are shown below. Released product was analysed by TLC (middle row) and sequencing gel (bottom row). Assays were repeated at least twice. CHES, MacroD1 and T. curvata PARG treatment of non-H-Y-E PARPS results in ADPr release, indicative of MAR synthesis activity. See also Supplementary Figs 4,5 . Full size image Most PARPs do not synthesize PAR upon automodification Incorporation reactions were performed on protein A magnetic beads using anti-GFP precipitation of the GFP–PARP fusions. Bead-bound GFP–PARPs were incubated with 5 or 10 μM NAD + supplemented with a constant ratio of 32 P-NAD + ( Fig. 1 ). Total NAD + concentrations were kept low to increase the ratio of hot:cold NAD + due to weak signal incorporation by many PARPs relative to PARP1 as identified during initial analysis. PARP1 exhibited robust polymer synthesis even at these low NAD + concentrations, indicating that NAD + is not limiting in our reactions ( Fig. 1 ). Several controls were performed to confirm that assay conditions did not affect PARP enzymatic activity. First we examined the effect of the N-terminal location of the GFP tag on PARP enzymatic activity by comparing the activity of both N and carboxy-terminal GFP fusions to PARP1. Both incorporated similar amounts of 32 P-ADPr, suggesting that the N-terminal location of the tag does not affect PARP enzymatic activity ( Supplementary Fig. 1a ), similar to published results for PARP10 using the similarly sized N-terminal TAP tag [14] . We examined the possibility that the presence of a tag itself affects PARP enzymatic activity by comparing NAD + incorporation of GFP–PARP10, SBP–PARP10 and untagged PARP10 ( Supplementary Fig. 1b ). These results show that the presence of the GFP fusion had no appreciable effect on PARP activity. Finally bead-bound GFP–PARP10 and soluble PARP10 exhibited similar enzymatic activity suggesting that performing the analysis on beads does not affect PARP activity ( Supplementary Fig. 1b ). Kleine et al. predicted PAR synthesis activity for H-Y-E containing PARPs. Consistent with this prediction and previously reported results, PARP1, 2, 5a and 5b incorporated ADPr in a manner consistent with PAR synthesis [15] , [40] , [41] , [43] ( Fig. 1 ). PARP1 and 2 automodification reactions contained additional signal that did not resolve in the SDS–PAGE gel and instead remained in the well, potentially due to branching, or very long polymer length ( Fig. 1 ). In contrast to predictions by Kleine et al. , the H-Y-E containing PARP3 and 4 incorporated ADPr in a pattern indicative of MAR synthesis, consistent with previously published reports for full-length PARP3 (ref. 45 ) and bacterially expressed PARP4 catalytic domain [42] . PARP4 is a component of the cytoplasmic Vault complex, and the ADP-ribosylation activity of purified Vault complexes containing PARP4 suggests that it can generate PAR [42] . Thus PARP4 could exhibit PAR synthesis activity when bound to Vault proteins, or the PAR activity found in Vault complexes could be due to other co-purifying PARPs. Interestingly, the Coomassie stain for GFP–PARP4 shows a single band at ~200 kDa; however, additional lower molecular weight signal was identified on the autoradiogram. This signal is likely due to a C-terminal cleavage product of GFP–PARP4 since the N-terminal GFP fusion is detectable at that molecular weight via anti-GFP blot, whereas an antibody raised against the very C terminus of PARP4 does not detect the lower molecular weight band ( Supplementary Fig. 2 ). PARP6, 7, 8, 10, 11, 12, 14, 15 and 16 each incorporated ADPr in a manner consistent with MAR synthesis ( Fig. 1 ). Identification of MAR activity for PARP7, 10, 12, 14, 15 and 16 is consistent with previously published reports [13] , [14] , [22] , [26] , [47] . Interestingly, PARP15 exhibited weak automodification activity instead strongly modifying a co-precipitating protein. This result suggests that in contrast to other PARPs, PARP15 is not a major target of its own enzymatic activity. PARP9 failed to incorporate detectable amounts of ADPr, suggesting that it is catalytically inactive, in agreement with previous reports ( Fig. 1 ) [44] . Very weak NAD + incorporation was observed for both isoforms of PARP13, predicted to be inactive due to the presence of a Q-Y-V catalytic motif for PARP13.1, and the lack of a catalytic domain for PARP13.2 (refs 14 , 50 ). Previous reports on the activity of bacterially purified PARP13 catalytic domain did not detect any NAD + incorporation [14] and our results are consistent with this ( Supplementary Fig. 3 ). Instead the weak incorporation identified in PARP13 purified from 293F cells could be due to activity of a sub-stoichiometric co-purifying PARP. The majority of PARPs are mono(ADP-ribosyl)ases To further confirm ADP-ribosylation activity, in vitro automodified PARPs were treated with enzymes specific for PAR or MAR hydrolysis or chemicals known to release ADPr from proteins at the site of protein linkage. The signal that remained attached to the PARP was then examined by resolving on SDS–PAGE followed by autoradiography, and the released reaction products examined by TLC or high-resolution TBE–polyacrylamide sequencing gels capable of resolving single units of ADPr ( Figs 2 , 3 ). Each assay was performed a minimum of two times and the results were highly concordant. PAR hydrolysis was analysed using Thermomonospora curvata poly(ADPr) glycohydrolase ( T. curvata PARG) treatment, which hydrolyses PAR chains, releasing ADPr as a product [48] . There have been conflicting reports on the ability of PARG to hydrolyse proximal ADPr–protein linkages or MAR [14] , [48] , [51] . Under our reaction conditions, we did not observe substantial signal release from automodified PARP1 E988Q , shown to generate only MAR modifications, suggesting that T. curvata PARG does not hydrolyse MAR to a significant extent, although a few exceptions are described below ( Supplementary Fig. 4a ) [29] . MAR hydrolysis was analysed using MacroD1 and terminal (ADPr) glycohydrolase (TARG1) [36] , [52] , [53] . Both enzymes hydrolyse MAR; however, although MacroD1 has no known activity on PAR [51] , [53] , [54] , TARG1 can release PAR chains through hydrolysis at the proximal ADPr–protein linkage, but cannot hydrolyse released polymers to ADPr [36] . We first verified that the hydrolysis activity of T. curvata PARG, MacroD1 and TARG is not affected by their substrate being bead bound by comparing hydrolysis of bead bound automodified GFP–PARP10 or SBP–PARP10 to soluble PARP10 ( Supplementary Fig. 4b ). There was no effect of bead binding on hydrolysis activity. To identify an appropriate enzyme concentration for the reactions, automodified GFP–PARP10 was treated with increasing amounts of TARG1, MacroD1 and T. curvata PARG ranging from 50nM to 500nM ( Supplementary Fig. 4c ). We also directly compared TARG1 and MacroD1 hydrolysis activity on automodified PARP1, 7, 10 and 14 ( Supplementary Fig. 4d ). Hydrolysis activity of both enzymes was comparable, and we chose MacroD1 for our subsequent analyses to minimize the possibility of reactivity to PAR ( Supplementary Fig. 4d ). For all analyses, treatment with the same concentrations catalytically inactive mutants of T. curvata PARG, TARG and MacroD1 did not result in significant hydrolysis of ADPr modifications and were used as controls ( Supplementary Fig. 4a–d ). Several chemicals have been identified that specifically cleave ADPr–protein linkages, releasing intact ADPr modifications [55] . Three were tested: 2-(cyclohexylamino)ethanesulphonic acid (CHES), pH9, hydroxylamine, pH 7.5 and sodium hydroxide, pH12 ( Fig. 4 ). Although CHES and NaOH treatment showed similar amounts of PAR release from in vitro automodified PARP1, NaOH resulted in degradation of free ADPr to AMP, consistent with previous reports [56] . We were unable to obtain substantial release of intact PAR upon neutral hydroxylamine treatment of PARP1, previously shown to result in robust release of carboxylate–ADPr linkages [55] ( Fig. 4 ). Therefore, CHES treatment was utilized for subsequent assays due to its ability to release ADPr from both acidic and lysine residues, allowing for the identification of ADPr modifications from both chemical linkages [55] . 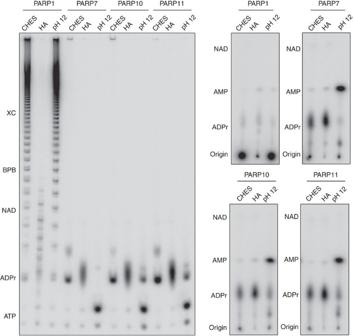Figure 4: Comparison of chemical treatments to release ADPr linkages. Automodified PARP1, 7, 10 and 11 were treated with 100 mM CHES, pH9, 2 mM EDTA or 0.4 M hydroxylamine, pH 7.5, 2 mM EDTA or 100 mM Tris, pH12, 1 mM EDTA. Released products were analysed both on 20% TBE–polyacrylamide sequencing gels (left) and TLC (right). Hydroxylamine treatment does not release PAR ladders from PARP1 and high pH treatment results in the degradation of ADPr to AMP. Figure 4: Comparison of chemical treatments to release ADPr linkages. Automodified PARP1, 7, 10 and 11 were treated with 100 mM CHES, pH9, 2 mM EDTA or 0.4 M hydroxylamine, pH 7.5, 2 mM EDTA or 100 mM Tris, pH12, 1 mM EDTA. Released products were analysed both on 20% TBE–polyacrylamide sequencing gels (left) and TLC (right). Hydroxylamine treatment does not release PAR ladders from PARP1 and high pH treatment results in the degradation of ADPr to AMP. Full size image PARP1 and 2 contain DNA binding domains, and their enzymatic activity is highly upregulated upon addition of DNA [41] , [57] . PARP3 does not contain a defined DNA binding domain; however, it was recently shown to bind and to be activated by DNA [46] , [58] . Our initial analyses of PARP3 activity identified low enzymatic activity in the absence of DNA to a point where the enzymatic activity of PARP3 was difficult to discern above background. Therefore, we compared the activity of GFP–PARP1–3 in the absence or presence of DNA ( Fig. 5 ). Automodification activity of all three PARPs was highly increased in the presence of DNA, consistent with previous results. In contrast, addition of DNA to PARP10 automodification reactions resulted in a slight decrease in activity ( Fig. 5 ). Addition of DNA to the PARP3 reactions did not change its reaction product—PARP3 still resolved as a distinct band consistent with MAR synthesis, indicating that ADPr synthesis activity is not altered upon upregulation of PARP enzymatic activity. Because addition of DNA to incorporation reactions increases activity without altering the pattern of NAD + incorporation, PARPs1–3 were automodified in the presence of DNA for TLC and sequencing gel analysis. 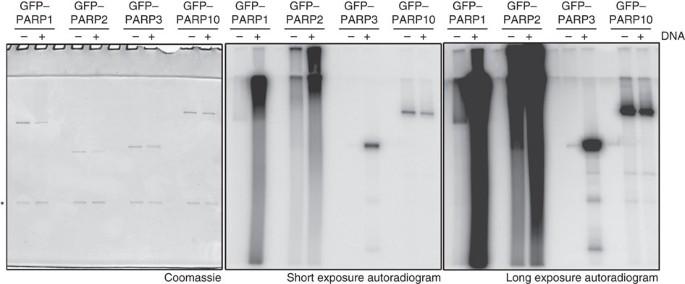Figure 5: DNA dependence of PARP enzymatic activity. GFP–PARPs 1, 2, 3 and 10 were immunoprecipitated from 293F cells and subjected to NAD+incorporation reactionsin vitrowith 10 μM cold NAD+supplemented with a constant ratio of 32P-NAD+, with or without the addition of activated DNA. Automodified PARPs were resolved on SDS–PAGE gels and subjected to Coomassie staining and autoradiography. Addition of DNA to PARPs 1, 2 and 3 results in upregulation of enzymatic activity whereas PARP10 activity is slightly decreased. Asterisk indicates IgG used for immunoprecipitation. Figure 5: DNA dependence of PARP enzymatic activity. GFP–PARPs 1, 2, 3 and 10 were immunoprecipitated from 293F cells and subjected to NAD + incorporation reactions in vitro with 10 μM cold NAD + supplemented with a constant ratio of 32P-NAD + , with or without the addition of activated DNA. Automodified PARPs were resolved on SDS–PAGE gels and subjected to Coomassie staining and autoradiography. Addition of DNA to PARPs 1, 2 and 3 results in upregulation of enzymatic activity whereas PARP10 activity is slightly decreased. Asterisk indicates IgG used for immunoprecipitation. Full size image Results for H-Y-E PARPs are shown in Fig. 2 and summarized in Table 1 . CHES treatment of the H-Y-E PARPs 1, 2, 5a and 5b resulted in release of PAR, seen as ladders on high-resolution DNA sequencing gels ( Fig. 2 ). T. curvata PARG treatment hydrolysed these PAR chains, causing the SDS–PAGE signal for each to collapse to distinct bands at their respective molecular weight, releasing ADPr as the major product as detected by TLC ( Fig. 2 ; see Supplementary Fig. 4e for migration patterns of cold and hot standards on TLC). Sequencing gel analysis of the released T. curvata PARG product showed that some short ADPr oligomers remained ( Fig. 2 ), consistent with previous data demonstrating that T. curvata PARG has lower activity on short PAR chains [59] . Finally, although MacroD1 did not cause a similar collapse of automodification signal to distinct band, treatment resulted in some release of PAR chains for PARPs 1, 2, 5a and 5b ( Fig. 2 ). Treatment with MacroD1 and T. curvata PARG catalytic dead mutants had no effect on the ADPr modifications. In contrast, CHES, MacroD1 and T. curvata PARG treatment of H-Y-E PARPs 3 and 4 resulted in the release of ADPr seen on both TLC and sequencing gel ( Fig. 2 ), similar to what was observed for H-Y-(I/L/Y) PARPs (below, Fig. 3 ). Since T. curvata PARG treatment resulted in minor ADPr release for PARP3 and 4, we confirmed that they contain attached MAR by treating with increasing amounts of bovine PARG using automodified PARP1 and PARP10 as controls ( Fig. 6 ). Bovine PARG treatment of PARP3, 4 and 10 had no effect on the ADPr signal attached to the protein whereas a dose-dependent loss of ADPr signal was identified for PARP1. Together, these results identify MAR synthesis activity for PARPs 3 and 4 ( Fig. 6 ). Table 1 Summary of PARP enzymatic activity. 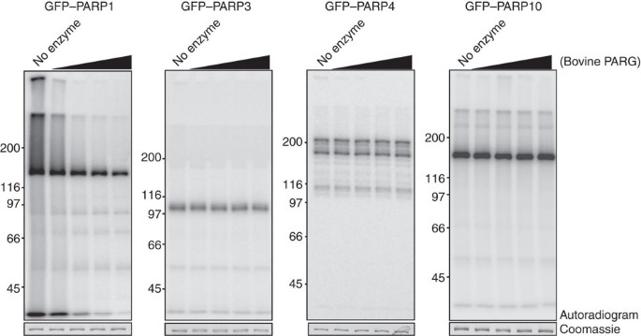Figure 6: Bovine PARG treatment of poly and mono(ADP-ribosyl)ating PARPs. Automodified GFP–PARPs 1, 3, 4 and 10 were treated with a titration of bovine PARG ranging from 1–10 ng ml−1. GFP–PARP1, which produces PAR, is sensitive to bovine PARG treatment whereas GFP–PARPs 3, 4 and 10, which produce MAR, do not show any decrease in signal upon bovine PARG treatment. Assay was repeated twice. Full size table Figure 6: Bovine PARG treatment of poly and mono(ADP-ribosyl)ating PARPs. Automodified GFP–PARPs 1, 3, 4 and 10 were treated with a titration of bovine PARG ranging from 1–10 ng ml −1 . GFP–PARP1, which produces PAR, is sensitive to bovine PARG treatment whereas GFP–PARPs 3, 4 and 10, which produce MAR, do not show any decrease in signal upon bovine PARG treatment. Assay was repeated twice. Full size image Results for non H-Y-E PARPs are shown in Fig. 3 and summarized in Table 1 . H-Y-(I/L/Y) PARPs exhibited release of ADPr as the major product of CHES and MacroD1 treatment ( Fig. 3 ). Treatment with T. curvata PARG also resulted in release of ADPr for some of these PARPs (albeit to a lesser extent than MacroD1 treatment), suggesting that some of the mono(ADP-ribosyl)ated sites might be sterically accessible for cleavage with the bacterial enzyme. ( Fig. 3 and Supplementary Fig. 5 ). The minor signal present at 2 units of ADPr for CHES treatment for many of the non-H-Y-E PARPs might be due to artifact, as it was also identified for PARP1 E988Q , although it is possible that this mutant could also synthesize short oligomers not previously detected ( Supplementary Fig. 5 ). In addition, increased background signal was observed for PARP4 and 16, possibly due to low incorporation activity under these conditions. Together, these results suggest that the primary activity of the H-Y-(I/L/Y) PARPs is mono(ADP-ribosyl)ation. The donor and acceptor loops impact enzymatic activity Our results identifying PARP3 and 4 as MARylating enzymes suggested that the simple presence of the H-Y-E motif is not sufficient to determine PAR synthesis—other structural elements must also be important. Since it has been postulated that the D-loop is an important structural component of the NAD + binding pocket [30] , we examined the D-loops of the H-Y-E PARPs. In addition, we examined their acceptor loops since they are thought to bind to elongating ADPr and protein targets and could therefore help determine the type of ADPr modification generated [31] . It is possible that the lack of PAR activity for PARP3 is due to the structure of its D-loop since this loop is a major structural difference between the PARP3 and PARP1 and 2 catalytic domains. The PARP1 D-loop contains three proline residues to contribute to loop rigidity whereas PARP3 only has one ( Supplementary Fig. 6 ). In addition, PARP3 lacks a tyrosine residue present in PARP1 that interacts with substrate, potentially affecting its ability to bind NAD + ( Supplementary Fig. 6 ) [60] , [61] . Together, this suggests that structural features of the D-loop can impact catalytic activity and that the presence of H-Y-E is not the sole indicator of PAR activity. The acceptor site is partially lined by the loop between β sheets 4 and 5 of the PARP catalytic domain and is thought to be important for substrate recognition [14] , [31] , [32] . Differences in amino acids lining the acceptor pocket are suggested to effect the type of ADPr that can be generated [61] and the acceptor loop length is specifically implicated in determining PARP catalytic activity [14] . Therefore, we tested its impact on enzymatic activity or the type of modification that can be generated. We tested the importance of the D-loop and acceptor loop on PARP1 enzymatic activity by assaying NAD + incorporation activity of PARP1/PARP16 chimeras in which either the donor or acceptor loops were swapped ( Fig. 7a ). The PARP16 D-loop was specifically chosen since it lacks prolines and is presumed to be relatively flexible, is not homologous to PARP1–3 D-loop sequence, and comes from a PARP with low MAR-generating activity (see discussion). PARP1 P16 D-loop no longer generated PAR and instead exhibited MAR synthesis activity, similar to what was previously shown for PARP1 catalytic glutamate point mutants [29] , confirming the importance of the D-loop on enzymatic activity ( Fig. 7a ). In contrast PARP1 P16 A-loop synthesized polymer, although incorporation activity was greatly reduced ( Fig. 7a ). This highlights the importance of the acceptor loop to PARP enzymatic activity and is consistent with a function for the acceptor pocket in binding of the terminal ADPr unit to be elongated by PARP1. 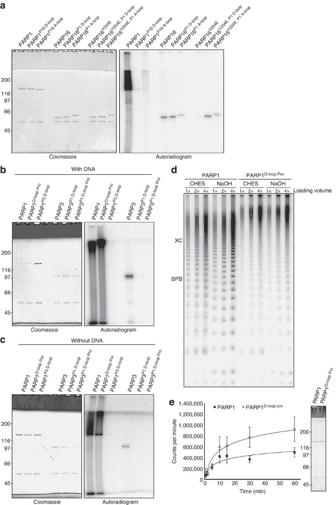Figure 7: Impact of donor and acceptor loops on enzymatic activity. (a) Wild-type and chimeric GFP–PARP1 and 16 constructs were expressed in 293F cells, immunoprecipitated and subject toin vitroNAD+incorporation assays. Assays were repeated twice. Replacement of PARP1 D-loop with PARP16’s (PARP1P16 D-loop) inhibited PAR synthesis activity instead resulting in MAR synthesis. In contrast replacement with the acceptor loop of PARP16 (PARP1P16 A-loop) retained PAR synthesis, but decreased total PAR activity. PARP16 activity was unchanged after replacement with either the PARP1 donor or acceptor loop. In contrast, PARP16Y254Einhibits the endogenous MAR synthesis activity that is restored by replacement with either the donor or acceptor loops of PARP1. (b,c) Wild type, PARP1D-loop Proand chimeric GFP–PARP1 and 3 constructs were expressed in 293F cells, immunoprecipitated and subject toin vitroNAD+incorporation assays either with (b) or without (c) DNA. Assays were repeated twice. Mutation of the three proline residues in the PARP1 D-loop results in an enrichment for PAR that resolves higher on the SDS–PAGE gel whereas replacement with the PARP3 D-loop results in MAR synthesis activity in the absence and presence of DNA. The GFP-PARP3P1 D-loopconstruct is not active. (d) Wild-type GFP-PARP1 and GFP-PARP1D-loop Prowere automodified and attached PAR chains were released with either CHES or NaOH and analysed by sequencing gel. Assay was repeated twice. GFP-PARP1D-loop Prois enriched for longer polymer. (e) NAD+incorporation kinetics of wild-type GFP-PARP1 and GFP-PARP1D-loop Proindicate that, although both proteins have similar initial reaction rates, the PARP1D-loop Proincorporation reaction does not plateau with similar kinetics,n≥3, error bars represent s.d., data fit to logarithmic regression. Representative Coomassie stain of input shown to right. See alsoSupplementary Figs 6,7. Figure 7: Impact of donor and acceptor loops on enzymatic activity. ( a ) Wild-type and chimeric GFP–PARP1 and 16 constructs were expressed in 293F cells, immunoprecipitated and subject to in vitro NAD + incorporation assays. Assays were repeated twice. Replacement of PARP1 D-loop with PARP16’s (PARP1 P16 D-loop ) inhibited PAR synthesis activity instead resulting in MAR synthesis. In contrast replacement with the acceptor loop of PARP16 (PARP1 P16 A-loop ) retained PAR synthesis, but decreased total PAR activity. PARP16 activity was unchanged after replacement with either the PARP1 donor or acceptor loop. In contrast, PARP16 Y254E inhibits the endogenous MAR synthesis activity that is restored by replacement with either the donor or acceptor loops of PARP1. ( b , c ) Wild type, PARP1 D-loop Pro and chimeric GFP–PARP1 and 3 constructs were expressed in 293F cells, immunoprecipitated and subject to in vitro NAD + incorporation assays either with ( b ) or without ( c ) DNA. Assays were repeated twice. Mutation of the three proline residues in the PARP1 D-loop results in an enrichment for PAR that resolves higher on the SDS–PAGE gel whereas replacement with the PARP3 D-loop results in MAR synthesis activity in the absence and presence of DNA. The GFP-PARP3 P1 D-loop construct is not active. ( d ) Wild-type GFP-PARP1 and GFP-PARP1 D-loop Pro were automodified and attached PAR chains were released with either CHES or NaOH and analysed by sequencing gel. Assay was repeated twice. GFP-PARP1 D-loop Pro is enriched for longer polymer. ( e ) NAD + incorporation kinetics of wild-type GFP-PARP1 and GFP-PARP1 D-loop Pro indicate that, although both proteins have similar initial reaction rates, the PARP1 D-loop Pro incorporation reaction does not plateau with similar kinetics, n ≥3, error bars represent s.d., data fit to logarithmic regression. Representative Coomassie stain of input shown to right. See also Supplementary Figs 6,7 . Full size image Replacement of the PARP16 donor or acceptor loops with those from PARP1 did not change the MAR activity of PARP16, although PARP16 P1 A-loop exhibited decreased enzymatic activity ( Fig. 7a ). Replacement of the tyrosine from the catalytic residues with glutamate completely abolished activity, similar to what was previously shown for PARP10 (ref. 14 ). Interestingly, substituting either the donor or acceptor loop of PARP1 in PARP16 Y254E restores MAR synthesis activity, indicating the primary sequence of the catalytic residues are not the sole determinant of enzymatic activity ( Fig. 7a ). Because the D-loop appeared to have the greatest impact on enzymatic activity, altering the nature of the modification generated by PARP1, we further investigated its contribution to ADPr synthesis. To do so, we generated PARP1/PARP3 chimeras in which the D-loops were swapped, and a PARP1 mutant in which the three proline residues of the D-loop (P881, P882, P885) were mutated to alanines (PARP1 D-loop Pro ) ( Fig. 7b,c ). We first examined enzymatic activity using fixed concentrations of 32 P-NAD + (10 μM) in the presence and absence of DNA. PARP1 D-loop Pro still had PAR synthesis activity in both conditions, although the pattern of incorporation differed from wild-type PARP1. Higher molecular weight product appeared to dominate the reaction product in PARP1 D-loop Pro reactions regardless of the reaction conditions ( Fig. 7b,c and Supplementary Fig. 7a , see below). In contrast, the PARP1 P3 D-loop no longer generated PAR and instead exhibited MAR synthesis activity consistent with results from the PARP1 P16 D-loop chimera ( Fig. 7a–c ). Because of the high level of PAR synthesis for wild-type PARP1 and PARP1 D-loop Pro in the presence of DNA, the Coomassie signal appears weaker due to smearing of the signal ( Fig. 7b ). In contrast, since PARP1 P3 D-loop resolves as a distinct band, the Coomassie signal is much stronger ( Fig. 7b ). Unlike the PARP16 chimera, the PARP3 P1 D-loop was inactive. These results suggest that simple replacement with a PAR competent D-loop is not sufficient for PAR synthesis activity ( Fig. 7a–c ). To determine if a similar pattern of PAR synthesis occurs for PARP1 D-loop Pro at physiological NAD + levels, we assayed product formation at increasing concentrations of NAD + substrate that include higher, more physiological concentrations of NAD + ( Supplementary Fig. 7b ). This analysis was done in the absence of DNA since our initial results indicated that the lower activity of the both PARP1 and PARP1 D-loop Pro highlighted the difference in the pattern of incorporation. At all NAD + concentrations PARP1 D-loop Pro reactions were enriched for PAR resolving at higher MW relative to wild type, confirming that this enrichment is due to the inherent enzymatic activity of the PARP1 D-loop Pro ( Supplementary Fig. 7b ). Two possibilities could result in the higher MW PAR found in the PARP1 D-loop Pro : an increase in branching, which has been suggested to contribute to high molecular weight PAR [41] , and the synthesis of longer polymer. To test for differences in the levels of branching, we treated automodified wild type and PARP1 D-loop Pro with phosphodiesterase I and analysed the released products via 2D-TLC ( Supplementary Fig. 7c ). The (PR) 2 AMP to PRAMP signal ratio found in wild type and PARP1 D-loop Pro were similar, suggesting that there was no difference in branching between the two products. To test for differences in polymer length, PAR synthesized by wild-type PARP1 and PARP1 D-loop Pro was analysed by resolving CHES and NaOH released product on TBE sequencing gels ( Fig. 7d ). CHES release was incomplete, with the unreleased product for the PARP1 D-loop Pro samples highly enriched for high molecular weight PAR ( Supplementary Fig. 7d ). PAR released from PARP1 D-loop Pro reactions exhibited a higher molecular weight distribution relative to wild type for both CHES and NaOH as analysed by TBE gel analysis suggesting that they contained longer polymers ( Fig. 7d ). To better understand the reaction product generated by PARP1 and PARP1 D-loop Pro , kinetic analysis was performed ( Fig. 7e ). Wild-type PARP1 and PARP1 D-loop Pro incorporated NAD + with similar kinetics at early time points (1–5 min); however, at later time points (including 30 min when samples shown on Fig. 7d were obtained) when the incorporation kinetics of PARP1 plateaued, PARP1 D-loop Pro incorporation continued to increase, consistent with the hypothesis that the higher molecular weight product results from generation of longer PAR polymers ( Fig. 7e ). Amino-acid specificity of PARP ADP-ribosylation reactions PARP1 has been shown to modify acidic residues and lysines [34] , [35] , [36] , [37] , [38] , [39] . Because differences in the structures of the acceptor pockets or other structural or enzymatic differences that exist between MAR versus PAR generating PARPs could impact which amino acids are targeted for modification, we determined if MAR-generating PARPs exhibit similar aa target selectivity. To do so, we examined PARP3, 6, 9, 10, 11, 12 and 16 automodification reactions using mass spectrometry ( Table 2 and Supplementary Table 2 ). PARP3 was specifically examined since it contains H-Y-E but only makes MAR. Our data identify glutamate and aspartate residues as the most commonly targeted amino acids for modification, especially for PARP3. Many preparations also contained modifications on lysine ( Table 2 ) consistent with previously published results for PARP1, although we cannot rule out the possibility that non-enzymatic chemical ligation is responsible for modifications at these sites, a known phenomenon [62] . Table 2 ADP-ribosylation sites identified by mass spectrometry analysis of automodified PARPs. Full size table Surprisingly, we also identified ADP-ribosylated cysteines in PARP 6, 8, 11 and 12 samples. Interestingly, although multiple clustered ADP-ribosylated cysteine residues were identified in PARP8, no modifications of acidic residues or lysines were detected, although this does not imply that they are not present. Furthermore, these modifications occurred in the PARP6/8-specific cysteine-rich domain that precedes the catalytic domain. Altogether, these observations may suggest that cysteine could be modified by some of the MAR-generating PARPs. However, as cysteine modifications were identified before adding exogenous NAD + , it is also possible that MAR-cysteine modification is due to the activity of other enzymes present in the human cell extracts ( Supplementary Table 2 ). To determine if the cysteine modifications were dependent on PARP activity, all four cysteines identified as ADP-ribosylated in PARP8 (C332, C367, C376, C395) were mutated to alanines and automodification reactions were performed for wild type and cysteine mutant GFP–PARP8 (PARP8 4A-C , Supplementary Fig. 8a ). An ~10–20% decrease in the amount of NAD + incorporated was identified for the cysteine mutant depending on the concentration of NAD + tested, suggesting that they are genuine sites of PARP8 automodification ( Supplementary Fig. 8a ). Additional unidentified modification sites are present in PARP8 as NAD + incorporation signal remained in the mutant ( Supplementary Fig. 8a ). NAD + incorporation was not observed using a catalytic dead point mutant of PARP8 (PARP8 H697A ), suggesting that the cysteine modifications are dependent on catalytic activity and are not due to non-enzymatic chemical ligation ( Supplementary Fig. 8b ). A large number of modification sites, mainly in PARP10 samples, occurred on the N terminus of peptides suggesting that they could be experimental artifact ( Supplementary Table 3 ). Although all the ADP-ribosylation peptides reported here have been identified very confidently, we are less confident about the precise localization of ADPr modifications at the sites reported in grey in Table 2 (the peptide N terminus of these peptides might be modified instead of the side chain of the internal residue) and they are therefore shown provisionally. In addition to cysteine, we detected ADP-ribosylation of three arginine residues on PARP10 ( Supplementary Table 3 ). As all three ADP-ribosylated arginines are the first residues of the peptide, the modification could occur either on the guanidine group (arginine side chain) or on the amino group (peptide N terminus). No sites were identified for PARP9 protein consistent with the known lack of catalytic activity of this protein. To systematically identify the enzymatic activity of each PARP protein, we performed multiple assays to accurately identify the reaction products for the entire family. Our data indicate that the major activity for most of the PARPs is mono(ADP-ribosyl)ation. We can now confidently ascribe MAR activity to the newly identified functions for PARPs in actin cytoskeletal regulation, membrane organelle regulation, signal transduction, the unfolded protein response, and the cytoplasmic stress response. This suggests that the mechanisms of PARP functions in these pathways are mediated by MAR modifications of target proteins, unless these PARPs function in an ADPr synthesis independent manner. Although the use of recombinant protein is standard in the PARP field, it is important to note that the use of recombinant proteins expressed as GFP-fusion proteins has potential limitations compared to analysis of endogenous protein. For instance, although the GFP tag had no effect on the enzymatic activity of PARP1 or PARP10 ( Supplementary Fig. 1 ), we cannot completely rule out the possibility that it does not affect the activity of other PARPs. However this systematic analysis would not have been possible without the use of recombinant protein as it enabled purification of large amounts of pure protein necessary for such analysis. Studies of MARylating PARPs have shown that trans substrates are also MAR-modified suggesting that automodification is a useful assay of activity [26] , [47] ; however, it is possible that some PARPs may have substrate-specific enzymatic activity not detected using automodification. Identifying the protein targets of MAR activity and identifying mechanisms of MAR function will be critical. The MAR activity exhibited by PARP3 and 4, coupled with the analysis of the PARP1/PARP3 and PARP1/PARP16 chimeras demonstrate the importance of the D-loop in the function of the catalytic domain. Its importance is further illustrated by the ability of the PARP1 D-loop chimera to restore PARP16 Y254E synthesis activity, suggesting that D-loop function can overcome deficiencies of H-Y-E motif mutants. The proline residues of the PARP1 D-loop have been proposed to provide structural rigidity [30] but the requirement for this rigidity in enzymatic activity had not been investigated. The mutation of the D-loop prolines to alanines resulted in an enzyme that generates longer polymer and has increased enzyme kinetics. This increase in polymer length produced by PARP1 D-loop Pro could be due to several factors including decreased self-regulation—automodification normally downregulates PARP1 enzymatic activity and this mechanism of self-regulation could be deficient in the PARP1 D-loop Pro mutant. Another possibility is an increase in the processivity of the enzyme since communication between the D-loop and the A-loop is possible. Regardless, our results suggest that the D-loop confers important regulatory information to the catalytic domain. Our results also suggest that the acceptor loop is important for the enzymatic activity of PARPs, but not the type of modification generated, since the PARP1 P16 A-loop chimera continued to generate PAR, albeit at lower levels. This is consistent with a function for the A-loop in the binding to substrate, either elongating polymer, or protein target. Consistent with results for PARP1, both acidic residues and lysines were identified as targets of MAR-generating PARPs suggesting that, in general, MAR and PAR generating PARPs modify similar amino acids. These results also argue that the sequence and structural constraints limiting PARPs to MAR synthesis, including the H-Y-E containing PARP3, do not affect their ability to modify canonical amino-acid targets. In contrast our identification of cysteine modifications suggest that MARylating PARPs may have the ability to modify a larger diversity of amino acids, although it remains to be determined if PARylating PARPs can also generate cysteine modifications. Why do cells need both types of ADPr modifications? MAR and PAR synthesis activities are both evolutionarily conserved, indicating that both have important functions in cellular physiology [63] . PAR functions during stress responses and physiological pathways that require the rapid assembly of multiprotein complexes, acting as a protein binding scaffold. The consequences of MAR modifications on target protein are less understood. Recent work showing that ADPr-binding Macro domain-containing proteins can specifically bind MARylated targets suggests that one function could be to regulate specific protein-protein interactions, similar to SH2 domains binding to phosphoproteins [17] , [23] , [64] . MAR modifications are also especially interesting because they could serve as primers for further elongation to PAR, with PARPs functioning cooperatively to synthesize polymer, allowing a cell to tightly regulate each step of PAR generation. This possibility is supported by in vitro data showing heterodimerization and activation of PARPs with distinct activities, by the fact that PARPs with each activity are localized in both the cytoplasm and nucleus and by the presence of multiple physiological protein complexes containing MAR and PAR generating PARPs [13] , [27] , [45] , [58] , [65] . A closer examination of MAR function, and a closer examination of the ability of MAR to initiate PAR polymerization will be important. Cell culture and reagents 293F cells (from ATCC) were grown at 37°/5% CO 2 in F17 media supplemented with 2% glutamax (Life Technologies). 32 P-NAD + was from Perkin Elmer. Bovine PARG and 10 × Activated DNA was from Trevigen. NAD + incorporation reaction GFP–PARPs or SBP–PARPs were expressed in 293F cells. Twenty-four to 48 h after transfection, cells were washed 3 × in ice-cold phosphate-buffered saline and lysed for 20 min on ice in cell lysis buffer (CLB, 50 mM HEPES, pH7.4, 150 mM NaCl, 1 mM MgCl 2 , 1 mM EGTA, 1 mM DTT, 1% Triton X-100, 1 μg ml −1 leupeptin, aprotinin, pepstatin, PMSF). Lysates were subject to ultracentrifugation at 100,000 g for 30 min. Cleared lysates were incubated for 1 h at 4 °C either with anti-GFP antibody (3E6, Life Technologies) pre-bound protein A magnetic beads (Millipore) or streptavidin sepharose (GE Healthcare Life Sciences). Beads were than washed 1 × 5 min in CLB, followed by 3 × 10 min washes in CLB containing 1 M NaCl, and 1 × 5 min wash in PARP reaction buffer (PRB; 50 mM Tris, pH 7.5, 50 mM NaCl, 0.5 mM DTT, 0.1% Triton X-100, 1 μg ml −1 leupeptin, aprotinin, pepstatin). Soluble PARP10 was produced by cleaving the SBP tag from immunoprecipitated SBP–PARP10 at PreScission protease sequence using HRV3C (Sigma-Aldrich). NAD + incorporation reactions were performed in PRB containing 10 μM NAD + (unless otherwise indicated) supplemented with 32 P-NAD at a 1:20 ratio for 30 min at 25 °C. For PARPs with low incorporation signals (PARP4, 5a and 16), NAD + incorporation was performed using a 1:5 ratio for 1 h at 25 °C for TLC and sequencing gel analysis of released products. For PARPs 1–3, activated DNA was added to NAD + incorporation reaction for TLC and sequencing gel analysis of released products. Following NAD + incorporation, beads were washed 6 × 5 min in PRB supplemented with 1 M NaCl, 100 μM NAD + and 10 μM ATP and 2 × 5 min in PRB containing 100 μM NAD + and 10 μM ATP. Beads were then resuspended in Laemmli sample buffer, heated to 65 °C for 10 min and run on 8% SDS–PAGE gels followed by autoradiography. For enzymatic and chemical treatments, beads were treated with indicated enzyme or chemical following NAD + incorporation and washes. MacroD1 was used at 0.5 μM and T. curvata PARG was used at 0.1 μM for 1 h at 25 °C. CHES release was performed for 2 h at 37 °C. Beads were then resuspended in Laemmli sample buffer and reaction supernatants were collected and either spotted on PEI-cellulose TLC plates (Macheray–Nagel) and resolved in 0.15 M LiCl/0.15 M formic acid or diluted 1:1 in PAR loading buffer (50% urea, 25 mM NaCl, 2 mM EDTA, 0.1% xylene cyanol, 0.1% bromophenol blue) and resolved on 20% polyacrylamide-TBE sequencing gels. For analysis of PARP1 D-loop Pro , NAD + titration was performed using a ratio of 0.75μCi hot NAD + :10 μM cold NAD + . For kinetic analysis, reactions were stopped using 20% TCA at indicated time points, incubated on ice for a minimum of 30 min, and spun at 16.1 K*g for 30 min at 4 °C. TCA pellets were washed with 5% TCA 3 times and treated with 0.5 ml 0.1N NaOH, 2% SDS at 37 °C overnight. Resuspended pellets were transferred to scintillation vials containing 5 ml of Emulsifier-Safe scintillation fluid (Perkin Elmer) and analysed by liquid scintillation counting. High pH release of PAR chains was performed in 0.1N NaOH, 20 mM EDTA at 60 °C for 2 h. Samples were neutralized with 0.1 N HCl and analysed by sequencing gels as described. PARP chimera generation GeneArt strings (Life Technologies) or G-blocks (IDT) were generated in which either the donor and acceptor loops of PARP’s 1, 3 and 16 were switched. See Supplementary Methods for amino-acid sequences that were switched. EcoRV (internal site)/SalI were used to clone PARP1 fragments into PARP1/eGFPC1, SbfI (internal site)/SalI were used to clone PARP3 fragments into PARP3/eGFPC1, and PstI (internal site)/SalI were used to clone PARP16 fragments into PARP16/eGFPC1. Constructs were expressed in 293F cells and used for NAD + incorporation assays as described above. Mass spectrometry analysis Streptavidin binding peptide tagged-PARP6, 8, 9, 10, 11 and 12 fusions were expressed in 293F cells and immunoprecipitated as described above. Following 3 × 10 min washes in 1 M NaCl/CLB, streptavidin sepharose beads were washed 2 × 5 min in PRB and proteins were eluted in 4 mM biotin/PRB for 1 h at 25 °C. PARP16 (1–273 AA) and PARP3 were purified with N-terminal His-tags in from Escherichia coli as previously described [66] . PARPs were incubated with 0.2 mM NAD + and ADP-ribosylated PARPs were digested with trypsin by using a modified FASP protocol [67] . The samples were solubilized in 8 M urea 100 mM Tris pH 8 and loaded on a centrifugal filter (Vivacon 500, 50 kDa MW cutoff, Sartorius Stedim Biotech). The low-molecular-weight components were removed by washing four times with 8 M urea. Urea was removed by washing four times with 100 mM ammonium bicarbonate and proteins were digested with trypsin (trypsin Gold, Promega, Madison, USA). Following overnight digestion, the resulting peptides were eluted from the filter by centrifugation and further recovered with two additional washes using 100 mM ammonium bicarbonate. The eluted peptides were dried in a vacuum centrifuge system (Vacufuge, Eppendorf, Hamburg, Germany) and resuspended in 40 μl 1% formic acid. The acidified peptide mixtures were analysed by nanoflow liquid chromatography tandem mass spectrometry (MS/MS) using a Q Exactive hybrid quadrupole-Orbitrap mass spectrometer (Thermo Scientific, Bremen, Germany). Following separation on a Thermo Scientific EASY-Spray PepMap C18 column (75 μm inner diameter × 50 cm, 2 μm particle size, 100 Å pore size) using an EASY-nLC 1000 UPLC system (Thermo Scientific, Odense, Denmark), peptides were injected into the mass spectrometer through a Thermo Scientific EASY-Spray ion source. Optimal loading amounts were experimentally determined by injecting 1 μl (1/40) of the sample using a 90-minute gradient (linear gradient from 0 to 22% acetonitrile for 60 min) and the samples were sequentially analysed multiple times using 150-minutes gradients (linear gradient from 0 to 22% acetonitrile for 120 min) and different mass spectrometric acquisition parameters (see below) to maximize the quality of MS/MS spectra. The Q Exactive was operated in the data-dependent mode to automatically switch between MS and MS/MS acquisition with the following general parameters: survey full MS spectra acquired with a m/z range of 300–1,800 Th, the resolution set to as value of 70,000 and AGC (automatic gain control) target value of 1,000,000 ions; dynamic exclusion of 40 s. In the ‘standard’ acquisition method up to 10 most intense ions were fragmented by higher-energy collisional dissociation with a maximum injection time of 60 ms, resolution of 17,500 and target value of 1,000,000. In addition, the samples were analysed by two highly sensitive acquisition methods both with a maximum injection time of 1,000 ms and resolution of 35,000. In the first highly sensitive method up to five most intense ions were fragmented and scanned with the target value of 500,000; for the second highly sensitive method, the most intense precursor ion was sequenced with the target value of 1,000,000. Raw data were combined and analysed with Andromeda-based MaxQuant (version 1.3.0.5) [68] . The search was performed the against UniProtKB human proteome (canonical and isoform sequences; downloaded in April 2013). Enzyme specificity was set to trypsin allowing for up to four missed cleavages. Methionine oxidation, protein N -acetylation and ADP-ribosylation (mass shift of 541.0611) on glutamate, aspartate, cysteine, arginine, lysine and on the peptide N terminus were set as variable modifications. MaxQuant was set up to automatically search for the following diagnostic ions in MS/MS spectra matched to ADP-ribosylated peptides: adenine (mass 135.0545), adenosine–H 2 O (mass 249.0862), adenosine monophosphate (AMP; mass 347.0631), ADP [69] . All reported fragmentation spectra were manually validated using stringent criteria (supplementary MS/MS spectra). Raw data (mzML format) and manually annotated spectra have been submitted to Peptide Atlas ( http://www.peptideatlas.org/ ), where they are available under the identifier PASS00485. Accession codes : Raw mass spectrometry data and manually annotated spectra have been deposited in Peptide Atlas ( http://www.peptideatlas.org/ ) under the identifier PASS00485. How to cite this article : Vyas, S. et al. Family-wide analysis of poly(ADP-ribose) polymerase activity. Nat. Commun. 5:4426 doi: 10.1038/ncomms5426 (2014).